New loci and coding variants confer risk for age-related macular degeneration in East Asians Age-related macular degeneration (AMD) is a major cause of blindness, but presents differently in Europeans and Asians. Here, we perform a genome-wide and exome-wide association study on 2,119 patients with exudative AMD and 5,691 controls, with independent replication in 4,226 patients and 10,289 controls, all of East Asian descent, as part of The Genetics of AMD in Asians (GAMA) Consortium. We find a strong association between CETP Asp442Gly (rs2303790), an East Asian-specific mutation, and increased risk of AMD (odds ratio (OR)=1.70, P =5.60 × 10 −22 ). The AMD risk allele (442Gly), known to protect from coronary heart disease, increases HDL cholesterol levels by 0.17 mmol l −1 ( P =5.82 × 10 −21 ) in East Asians ( n =7,102). We also identify three novel AMD loci: C6orf223 Ala231Ala (OR=0.78, P= 6.19 × 10 −18 ), SLC44A4 Asp47Val (OR=1.27, P =1.08 × 10 −11 ) and FGD6 Gln257Arg (OR=0.87, P= 2.85 × 10 −8 ). Our findings suggest that some of the genetic loci conferring AMD susceptibility in East Asians are shared with Europeans, yet AMD in East Asians may also have a distinct genetic signature. Age-related macular degeneration (AMD) is a progressive, blinding disease affecting millions of elderly individuals worldwide [1] , [2] . Several genome-wide association studies (GWAS) have identified common variants associated with AMD in European-ancestry populations [3] , [4] , [5] , [6] , and recently, rare genetic variation at CFH , CFI , C3 and C9 were also shown to strongly associate with AMD in Europeans [7] , [8] , [9] , [10] . However, there are few such studies in Asians [11] . Importantly, Asians appear to have a distinct clinical presentation of the disease (for example, absence of drusen and minimal fibrous scarring in polypoidal choroidal vasculopathy, a variant of AMD accounting for 20–55% of Asian patients with exudative AMD) and different responses to treatment (for example, poorer response to inhibitors of vascular endothelial growth factor (VEGF) compared with patients of European ancestry) [12] , [13] . It remains unclear whether there are differences in underlying genetic characteristics of AMD between patients of Asian versus European ancestry. Concurrently, previous GWAS studies provide limited coverage of low-frequency coding variants, which may result in the loss of function and are often ethnic-specific. There is thus interest in genetic studies of AMD and other diseases beyond standard-content GWAS to discover potentially causative coding variants in different ethnic groups. To address these questions, the Genetics of AMD in Asians Consortium perform a genome-wide (GWAS) and exome-wide association study (EWAS) of advanced AMD solely on the exudative (neovascular) disease subtype in East Asians. Compared with standard-content GWAS arrays, the exome array has significantly increased marker density across the coding human exome, thus increasing power to detect disease associations located within the coding frame. EWAS of AMD have not been previously conducted in either Europeans or Asians. In this paper, we present data from eight independent AMD case–control collections enrolled across multiple sites in East Asia, totalling 6,345 exudative AMD cases and 15,980 controls. This is the largest sample, to our knowledge, of East Asians ever assembled for genetic studies of AMD. 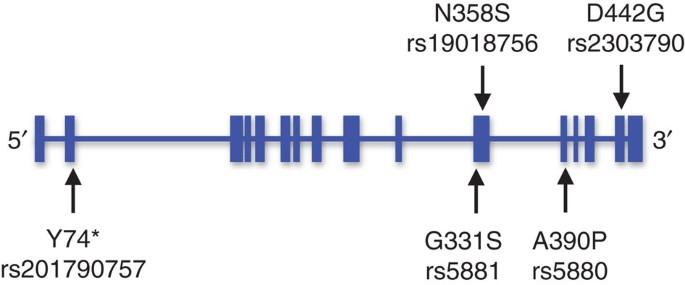Figure 1: Genomic organization of theCETPgene. The position of five rare (minor allele frequency <0.05) amino-acid changes observed in the discovery samples are shown as indicated by the arrows. Horizontal bars represent the position of exons in theCETPgene. Association with previously identified AMD variants After genotype imputation, synchronization and stringent quality filters were performed, a total of 4,471,719 SNPs were assessed for the GWAS and 120,027 autosomal coding-frame SNPs for EWAS from 2,119 AMD cases and 5,691 controls ( Table 1 ). Overall genomic inflation was very low ( λ gc =1.031; Supplementary Fig. 1 ), suggesting minimal confounding of the disease association analysis by population stratification or other systematic study design biases. Data from the discovery stage analysis confirmed previously identified AMD variants in ARMS2-HTRA1 rs10490924 ( P =1.20 × 10 −103 ), CFH rs10737680 ( P =7.54 × 10 −38 ), CETP rs3764261 ( P =1.66 × 10 −12 ), ADAMTS9 rs6795735 ( P =1.13 × 10 −5 ), C2 - CFB rs429608 ( P =1.06 × 10 −4 ), as well as CFI rs4698775 ( P =7.5 × 10 −4 ; Supplementary Table 1 and Supplementary Fig. 2 ). Our data also showed nominal evidence of replication in the same direction as the initial study for a further three previously reported variants ( TGFBR1 rs334353, APOE rs4420638, and VEGFA rs943080; P <0.05 for each). The remaining 8 out of 17 previously described SNPs that were non-monomorphic in our East Asian collections did not show evidence of replication in our study ( Supplementary Table 1 ). A recently described rare, functional and highly penetrant genetic mutation within CFI (G119R, rs141853578) shown to confer markedly elevated risk of AMD in Europeans [14] was observed to be non-polymorphic in our East Asian samples ( Supplementary Table 1 ). Similarly, recently described rare mutations in C3 (K155Q, rs147859257) and C9 (P167S, rs34882957) were also shown to be non-polymorphic in our East Asian samples ( Supplementary Table 1 ). Table 1 Baseline characteristics of exudative age-related macular degeneration cases and controls in the discovery and replication sample collections. 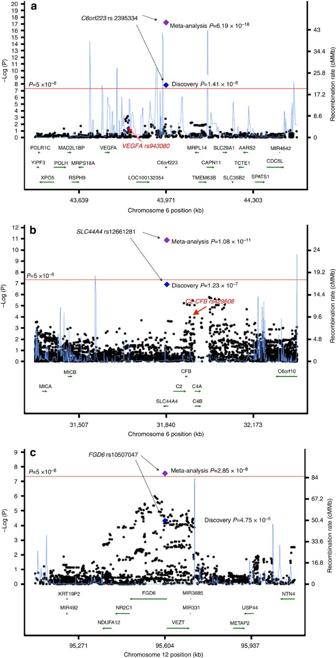Figure 2: Regional association plots at the three risk loci for exudative age-related macular degeneration. (a) TheC6orf223locus (rs2295334):VEGFArs943080, which is located in the intergenic, non-coding region, was very strongly associated with AMD in Europeans, but this study of exudative AMD in East Asians could not reveal significant association with it (P=0.041 by score-based tests using logistic regression in 2,119 cases and 5,691 controls). The two markers are independent from each other (r2=0.0), as well as separated by strong recombination events in Asians. (b) TheSLC44A4locus (rs12661281):C2-CFBrs429608 was very strongly associated with AMD in Europeans, but revealed modest evidence of association in our discovery stage (P=1.06 × 10−4). The two markers are independent from one another (r2=0.01). (c) TheFGD6locus (rs10507047). Full size table Discovery of new SNP variants associated with AMD Apart from verifying previous observations, our discovery analysis also revealed genome-wide significant association at C6orf223 (rs2295334 encoding for A231A, P =1.41 × 10 −8 ; Table 2 , Supplementary Table 2 and Supplementary Fig. 2 ), a novel SNP marker not previously reported to associate with AMD risk. We observed a further 21 independent SNPs from distinct loci not previously implicated with susceptibility to AMD showing evidence of association surpassing P <1 × 10 −4 . We then brought forward all the 22 markers ( Table 2 ) for replication genotyping in independent sample collections comprising 4,226 exudative AMD cases and 10,289 controls ( Table 1 ). Replication evidence was compelling for CETP rs2303790 (encoding D442G; odds ratio (OR)=1.73, P =2.95 × 10 −16 ), as well as for C6orf223 rs2295334 (A231A; OR=0.80, P =5.25 × 10 −11 ), SLC44A4 rs12661281 (D47V; OR=1.22, P =5.13 × 10 −6 ) and FGD6 rs10507047 (Q257R; OR=0.88, P =7.69 × 10 −5 ), leading to genome-wide significant findings in the meta-analysis of all 6,345 AMD cases and 15,980 controls ( P <5.0 × 10 −8 for each of the four loci; Table 2 and Supplementary Table 2 ). Genotyping clusters were directly visualized for the top SNPs and confirmed to be of good quality ( Supplementary Fig. 3 ). Table 2 Summary of results of the genome-wide and exome-wide association study on exudative age-related macular degeneration. Full size table Of note, we did not observe any substantial difference in the association signals of the most significant SNPs in the subgroup analysis of our AMD cases by typical neovascular AMD ( n =1,083 cases) and polypoidal choroidal vasculopathy ( n =1,015 cases; Supplementary Table 3 ). The effect size for each of the top SNPs was similar between the two AMD subgroups. Conditional analysis The presence of the mutant CETP 442G (rs2303790) allele is seen only in East Asians (for example, Chinese, Japanese and Koreans; minor allele frequency (MAF) <5% in our controls) and not in South Asians, Europeans or Africans. This mutation is independent from all previously described common, non-coding polymorphisms near the CETP locus ( r 2 <0.1; Supplementary Fig. 4 ). Regional association analysis conditioning on other known common AMD variants in CETP confirmed the independence of D442G from other nearby common variants ( Supplementary Tables 4 and 5 ). We also genotyped and assessed multiple, rare, protein-changing mutations at CETP , including Y74Stop, G331S, N358S and A390P ( Fig. 1 ). None of them showed association with AMD ( Table 3 ). Mutational load and haplotypic analysis considering all amino-acid changes within CETP confirmed that the D442G mutation drove all signals of association between CETP and AMD ( Table 4 ). Figure 1: Genomic organization of the CETP gene. The position of five rare (minor allele frequency <0.05) amino-acid changes observed in the discovery samples are shown as indicated by the arrows. Horizontal bars represent the position of exons in the CETP gene. Full size image Table 3 Single variant analysis (score-based tests using logistic regression) of the five observed CETP rare variants with exudative age-related macular degeneration in the discovery stage. Full size table Table 4 Results of association of the five observed CETP rare variants with exudative age-related macular degeneration using gene-based tests in 2,119 cases and 5,691 controls in the discovery stage. Full size table C6orf223 is located ~220,000 base pairs downstream of VEGFA and ~150,000 base pairs from rs943080, a marker previously shown to strongly associate with AMD in Europeans [5] , [6] . In this study of AMD in East Asians, the evidence of association for VEGFA rs943080 was only nominally significant ( P =0.041 in the discovery stage; Supplementary Table 1 ). Linkage disequilibrium analysis revealed no correlation between C6orf223 rs2295334 and VEGFA rs943080 ( r 2 =0.0), with both markers separated by significant recombination events ( Fig. 2a ). Logistic regression adjusting for the allele dosage at VEGFA rs943080 did not reveal any attenuation of the association signal for C6orf223 rs2295334 ( P =1.66 × 10 −8 ; Supplementary Table 6 ). Regional association analysis including all markers from the genome and exome array data conditioning on C6orf223 rs2295334 also did not reveal any secondary signal of association within its 1 Mb flanking region ( Supplementary Table 7 ), thus pointing to C6orf223 rs2295334 as a novel and uncharacterized genetic risk factor for exudative AMD in East Asians. Figure 2: Regional association plots at the three risk loci for exudative age-related macular degeneration. ( a ) The C6orf223 locus (rs2295334): VEGFA rs943080, which is located in the intergenic, non-coding region, was very strongly associated with AMD in Europeans, but this study of exudative AMD in East Asians could not reveal significant association with it ( P =0.041 by score-based tests using logistic regression in 2,119 cases and 5,691 controls). The two markers are independent from each other ( r 2 =0.0), as well as separated by strong recombination events in Asians. ( b ) The SLC44A4 locus (rs12661281): C2-CFB rs429608 was very strongly associated with AMD in Europeans, but revealed modest evidence of association in our discovery stage ( P =1.06 × 10 −4 ). The two markers are independent from one another ( r 2 =0.01). ( c ) The FGD6 locus (rs10507047). Full size image SLC44A4 is located ~116,000 base pairs away from a previously reported AMD locus, C2 - CFB (rs429608) [6] . Nevertheless, SLC44A4 rs12661281 has no correlation with C2-CFB rs429608 ( r 2 =0.01) and showed the strongest evidence of association with AMD within the genomic region ( Fig. 2b ), suggesting it to be also a new and uncharacterized risk factor for AMD. Logistic regression analysis adjusting for allele dosage at C2-CFB rs429608 did not result in any significant change in magnitude of the association either at SLC44A4 rs12661281, testifying to their mutual independence (OR unconditioned =1.38, P unconditioned =1.10 × 10 −7 ; OR conditioned for rs429608 =1.35, P conditioned for rs429608 =1.49 × 10 −6 ; Supplementary Table 8 ). Gene-based tests on mutational load We next proceeded to conduct gene-based tests on mutational load to further investigate the role of low-frequency variants in exudative AMD for all the patient collections in the discovery stage. Gene-based tests are an alternative to single-marker tests for association, which are often underpowered to detect association with rare variants. We performed our tests as previously described [15] . To more directly address the impact of low-frequency, non-synonymous genetic variants, we considered only 109,296 such variants with MAF <5%. As a result, we were able to assess a total of 10,736 genes having at least two such variants using the sequence kernel association optimal (SKAT-O) test [16] . We did not detect significant evidence of association ( P <5 × 10 −8 ) between mutational load and AMD at any of the 10,736 genes tested, which are consistent across all three discovery sample collections. Nonetheless, while looking up on previously reported 22 genes within 17 distinct loci ( Supplementary Table 1 ) associated with AMD in European populations, we note nominal evidence of association between genetic load at CETP ( P unconditioned =5.38 × 10 −6 ), whereby the association was almost entirely driven by D442G ( P conditioned for D442G =0.96; Table 4 ) as well as C2 and AMD ( P =1.83 × 10 −6 , Supplementary Table 9 ). All the observations exceeding P <1 × 10 −4 for gene-based tests on mutational load summarized across the three discovery collections are appended as Supplementary Table 9 . CETP 442G, HDL and coronary heart disease The mutant CETP 442G allele was shown to result in an abnormally functioning CETP protein [17] . As CETP is a critical component of the pathways that regulate high-density lipoprotein cholesterol (HDL-c) [18] , we assessed this mutation for associations with serum HDL-c levels using linear regression, with adjustment for age, gender and body mass index, in three population-based cohorts of Singaporean Chinese [19] , [20] , [21] and Japanese [22] ( n =7,102, see details on the study cohorts in Supplementary Methods ) where GWAS data were available. We noted a strong association between 442G allele and increased HDL-c levels ( β =0.174 mmol l −1 per copy of 442G allele; reflecting an ~10% shift within the normal HDL range, P =5.82 × 10 −21 ; Table 5 ). This effect size is at least twice that observed for other CETP variants reported in European populations ( Supplementary Table 10 ) [23] , [24] . Table 5 Association of serum HDL cholesterol level and CETP D442G in East Asian population-based cohorts. Full size table Due to its strong effect on serum HDL-c, we assessed whether the mutant CETP 442G allele conferred any effect on individual susceptibility to coronary heart disease (CHD) in East Asians. Using 683 CHD cases and 1,281 controls from the Singapore Chinese Health Study ( Supplementary Methods ) [25] , we noted some degree of enrichment of the HDL-increasing, mutant 442G allele in the controls (2.89%) compared with the cases (2.42%, OR=0.83), although this did not reach statistical significance ( P =0.39). However, our observations were consistent with a recent study from Japan which analysed CETP D442G in 4,399 CHD cases and 7,672 controls whereby enrichment of the 442G allele were also found in the controls (3.4%) compared with the CHD cases (2.8%; OR=0.83, P =0.02) [26] . We thus performed a meta-analysis of our study and the Japanese study, resulting in a consistent protective effect of this mutation with CHD (OR=0.83, P =0.011, I 2 =0.0%; Supplementary Fig. 5 ). Our studies of exudative AMD in East Asians identified three novel loci ( C6orf233 , SLC44A4 and FGD6 ), two of which ( SLC44A4 and FGD6 ) harbour coding, non-synonymous variants. These have not been identified in large samples of AMD patients of European descent [6] , thus validating the role of searching for coding variations in diverse ethnic groups to better understand mechanistic basis of complex diseases such as AMD. Our most interesting findings were the identification of an uncommon East Asian-specific mutation at CETP (D442G) associated with exudative AMD. The association is the strongest (per-allele OR=1.70) observed outside of the classical CFH and ARMS2 - HTRA1 loci in East Asians. A common variant (rs3764261) mapping to the intergenic region between HERPUD1 and CETP was previously linked to AMD in Europeans, yet its effect size was modest (OR=1.15) [5] and independent from the D442G association. The mutant 442G allele is known to impair CETP function with reduction in plasma CETP mass and activity [17] , [27] , and is associated with elevated HDL-c in Japanese families [17] , [27] . This allele is absent in European populations [28] and appears to be present only in East Asians, rendering it independent from all other previously described common, non-coding CETP polymorphisms. We showed that each copy of the dysfunctional 442G allele confers, on average, a rise in HDL-c levels of 0.174 mmol l −1 and confirmed findings from the earlier Japanese studies. Given the mean serum HDL-c concentration is 1.3 mmol l −1 , this is a mutation of considerable effect size even from a population-based perspective. Notably, no other amino-acid substitutions within CETP detected by our GWAS and EWAS showed any evidence of association with AMD ( Fig. 1 and Table 3 ), suggesting that the D442G mutation is a possible causative mutation of AMD in East Asians in the CETP locus. We are not surprised that CETP D442G did not show a clearly significant protective effect against CHD as increasing lines of evidence more directly implicate LDL as the driving force for CHD susceptibility [29] , [30] . C6orf223 is a newly mapped gene with yet unknown functional role. Its A231A synonymous coding change is fivefold rarer in Europeans (MAF=0.03) as compared with Asians (MAF >0.15, Supplementary Table 2 ). It is thus unsurprising that the European GWAS efforts have yet to detect this locus. VEGFA rs943080, a marker strongly associated with AMD in European-ancestry populations [5] , is in the vicinity of C6orf223 , but its association with AMD is much weaker in this study of East Asians ( Supplementary Tables 1 and 6 ), possibly reflecting the differences in therapeutic response to anti-VEGF treatment between Asians and Europeans [13] , [31] . The D47V mutation within SLC44A4 is not included in most of the routinely used genotyping arrays, but is now included as part of the exome array used in this study. The genomic region around the SLC44A4 locus is more complex, being located within the broad MHC region on Chromosome 6 between HLA class I and class II genes. As this region is very polymorphic, and allele frequency differences between cases and controls could be confounded by even minor population stratification, we thus reassessed the associations with AMD by adjusting for the first 10 principal components (PCs) of genetic ancestry. We did not observe any change in the association signals observed from our standard analysis, which adjusted for the first five PCs (analysis adjusting for the top 10 PCs; OR=1.39, P =2.33 × 10 −7 in the discovery phase), consistent with previous observations in Asian studies with well-replicated associations within the MHC region [32] , [33] . SLC44A4 encodes for choline transporter protein-4, involved in sodium-dependent choline uptake by cholinergic neurons [34] . Defects in SLC44A4 have been linked to sialidosis, which presents with a spectrum of symptoms including eye abnormalities [35] . Prior studies on the basis of European patient collections have identified a total of four distinct AMD-associated loci on Chromosome 6 alone [6] . In this light, the burden of proof for the positive identification of C6orf223 and SLC44A4 (both are also located on Chromosome 6) is higher than usual due to the need for appropriate considerations of previously reported variants on the same chromosome. It is reassuring to note that both C6orf223 and SLC44A1 showed the strongest two signals of association with AMD outside of CFH , ARMS2 - HTRA1 and CETP . Our exhaustive analyses using logistic regression adjusting for allele dosages at previously described SNP markers suggest that both C6orf223 and SLC44A1 are unrelated to those previously reported, and thus they likely represent Asian-specific genetic associations for AMD. Neither FGD6 nor the genes within its vicinity ( Fig. 2c ) have ever been previously implicated in any ocular disorders. FGD6 encodes for FYVE, RhoGEF and PH domain-containing protein 6, with its functions yet to be characterized. The Q257R mutation is less than half as common in Europeans (MAF=0.10) compared with East Asians (MAF=0.20–0.30), again possibly explaining the ability of our study to pick up this genetic effect. The identified genes were expressed in human retinal pigment epithelium ( Supplementary Table 11 ). Of the three non-synonymous substitutions, the CETP D442G variant was predicted by both PolyPhen [36] and SIFT [37] to likely be causing damage to the protein structure/function, the FGD6 Q257R variant was predicted only by PolyPhen to be probably damaging but by SIFT to be tolerated and the SLC44A4 D47V variant was predicted by both tools to be benign or tolerated. Although the use of both prediction algorithms has been reported to be moderately sensitive, they suffer from lack of specificity [38] , and thus more evidence should be sought with regards to the FDG6 and SLC44A4 non-synonymous variants. Using HaploReg [39] , RegulomeDB [40] and Encyclopaedia of DNA Elements (ENCODE) [41] data, we identified variants within each of the four LD blocks in the 1000 Genomes Project ( r 2 >0.8 and <250 kb from the top SNP) to apply functional annotations relevant to the regulation of transcription ( Supplementary Table 12 ). In addition to their functions on amino-acid substitutions, all of the four identified variants lie within a DNase I hypersensitivity site or in a region where modification of histones is suggestive of promoter, enhancer and other regulatory activity, and/or have an influence on binding of transcription factors or effects on a specific regulatory motif. C6orf223 A231A (rs2295334) and FGD6 Q257R could tag genetic variants that lie in potential transcription-factor binding sites ( Supplementary Table 13 ). Examination of a recently available large-scale eQTL mapping database [42] indicates that out of the four novel genome-wide significant SNPs, markers SLC44A4 D47V and FDG6 Q257R could serve as cis-eQTLs. The minor allele at SLC44A4 D47V (rs12661281) is associated with significantly altered expression of HSPA1B and CSKN2B, which are located within a 210,000 bp region flanking SLC44A4 D47V. The minor allele at FDG6 Q257R (rs10507047) is associated with significantly increased expression of the neighbouring VEZT gene ( Supplementary Table 14 ). Given that these findings are based on expression in whole blood in European samples, further work will be needed to elucidate their role in retinal tissue and in Asian samples. Nonetheless, these could suggest possible alternate mechanisms whereby both non-synonymous substitutions potentially affect AMD risk apart from directly affecting the protein structure of their parent genes. Our study examined mainly the exudative subtype of AMD, and therefore cannot be completely compared with other studies looking at advanced AMD including the choroidal neovascularization and geographic atrophy subtypes. We also note substantial differences in inter-ethnic MAF for most of the previously reported loci associated with AMD in European-ancestry populations ( Supplementary Table 1 ). This could represent genuine differences in genetic architecture in AMD between Asians and Europeans, or that the low allele frequency in either ethnicity could result in insufficient power to replicate genome-wide significant hits initially observed in either Asians or Europeans. Overall, out of 21 previously reported SNPs showing strong evidence of association in Europeans, we were able to replicate 9 of them in our study of East Asians at P <0.05. Taken together with the three novel loci and one novel variant in CETP in East Asians discovered in this study, we postulate that the genetic mechanisms of AMD in Asians could, in part, be somewhat distinct from that in Europeans. In summary, our genome-wide and exome-wide study of AMD provides new insights into the genetic mechanisms of AMD in East Asians. Our study highlights the value of searching for low-frequency, ethnic-specific genetic variants on the coding frame of AMD that may inform pathogenesis. Although some of the genetic loci conferring disease susceptibility in East Asians are shared with Europeans (for example, common variation mapping to CFH , HTRA1 and CETP ), we identified significant important differences in the fine-scale genetic architecture of AMD, which appear specific to East Asians. Such differences could underpin at least some of the inter-ethnic differences in clinical presentation and response to specific therapies, including the poorer response to anti-VEGF therapy in Asians. Study design and phenotyping We performed a GWAS and EWAS on neovascular AMD in East Asians. In the discovery stage, we included and genotyped 2,119 cases and 5,691 controls from three case–control studies from Singapore, Hong Kong and Japan. For replication, five independent case–control studies were conducted in Korea, Japan, and Guangdong, Sichuan and Beijing in China, totalling 4,226 cases and 10,289 controls. All the studies were performed with the approval of their local Medical Ethics Committee, and written informed consent was obtained from all the participants in accordance with the Declaration of Helsinki. A detailed description of subject recruitment and phenotyping in each sample collection is provided in Supplementary Methods , and summarized in Table 1 . In brief, the diagnosis of exudative AMD was made at each site by retinal specialists, according to standard clinical definitions on the basis of detailed ophthalmic examinations, including dilated fundus photography, fluorescein angiography, indocyanine green angiography and optical coherence tomography ( Table 1 ). Grading of fluorescein angiograms for the presence of choroidal neovascularization were performed using a modification from the Macular Photocoagulation Study [43] . Indocyanine green angiography was performed to diagnose definitive polypoidal choroidal vasculopathy, a variant of AMD, using the Japanese Study Group guidelines [44] . Cases with other macular diseases such as central serous chorioretinopathy, high myopia and angioid streaks were excluded. Of the 2,119 exudative AMD cases included in the discovery phase, 1,083 (51%) were classified as ‘typical neovascular AMD’, 1,015 (48%) were polypoidal choroidal vasculopathy and 21 (1%) had one eye with typical neovascular AMD and the other eye with polypoidal choroidal vasculopathy. At each site, controls subjects without any clinical signs of AMD were either recruited from eye clinics or enrolled from population-based studies ( Supplementary Methods ). Genotyping and imputation For the discovery stage, GWAS genotyping was performed using the Illumina Human OmniExpress or Human Hap610-Quad beadchips, and EWAS was done using HumanExome beadchips ( Table 1 ). For replication, genotyping was performed using the MassArray platform (Sequenom), as well as using Taqman allelic discrimination probes (Applied Biosystems). Stringent quality control filters were used to remove poorly performing samples and SNP markers in both the discovery and replication (de-novo genotyping) phases. For the GWAS, SNPs with a call rate of <95%, MAF of <1%, or showing deviation from Hardy–Weinberg Equilibrium ( P <10 −6 ) were removed from further statistical analysis. For the EWAS, SNPs with a call rate of <99%, MAF of <0.1% or showing deviation from equilibrium ( P <10 −6 ) were removed. The 99% threshold was used as many SNP markers on the exome array had MAF <5%, and as such, differential genotyping success rates between cases and controls as low as 2% could result in false-positive findings. SNPs which were not monomorphic (whereby at least one heterozygous carrier individual was present) were included for downstream analysis. Routine quality control criteria on a per-sample basis were carried out, and poorly performing samples were removed from further analysis. The remaining samples were then subjected to biological relationship verification by using the principle of variability in allele sharing according to the degree of relationship. Identity-by-state information was derived using the PLINK software [45] . For those pairs of first-degree relatives so identified (for example, parent–offspring, full-siblings, as well as monozygous twins), we removed the sample with the lower call rate before performing PC analysis. The imputation was carried out using IMPUTE2 version 2.2.2 with ASN population haplotypes from 1000 Genomes as reference, as described elsewhere [46] , [47] , [48] . Imputed genotypes were called with an impute probability threshold of 0.9 with all other genotypes classified as missing. Additional quality control filters were applied to remove SNPs with >1% missingness should the SNP have a MAF <5% in either cases or controls. For common SNPS with MAF >5%, the filtering criteria were set at >5% missingness. Statistical analysis For the discovery stage, all exudative AMD cases and controls appear well matched when visualized spatially on PC analysis for each sample collection on a per-country basis for Hong Kong, Japan and Singapore and according to self-reported ethnicity (ethnic Chinese for Hong Kong and Singapore, and ethnic Japanese for Japan; Supplementary Fig. 6 ), using previously reported criteria [49] , indicating that population stratification is unlikely to confound the association results. For both the discovery and replication stages, analysis of association with exudative AMD was carried out using 1-degree of freedom score-based tests using logistic regression. The tests model for a trend-per-copy effect of the minor allele on disease risk. For the discovery stage, we incorporated the top five PCs of genetic stratification into the logistic regression model to minimize the effect of residual population stratification [50] . We could not adjust for population stratification for the replication stage due to limited number of SNPs tested. Meta-analysis was conducted using inverse variance weights for each sample collection, which calculates an overall Z-statistic, corresponding P value and accompanying per-allele OR for each SNP analysed. Gene-based tests on mutational load was performed using the SKAT-O test [16] . The association between CETP D442G and serum HDL-c level was assessed using linear regression assuming an additive model of inheritance as previously described [23] (due to serum HDL-c being distributed normally), with adjustment for age, gender and body mass index. Regional association and PC plots were analysed and plotted using the R statistical software package. Power calculations For the discovery stage (2,119 AMD cases and 5,691 controls), power calculations [51] indicated that there is 80% power of detecting loci at P <1 × 10 −4 (the threshold of association for bringing forward SNPs to the replication stage) at MAF as low as 10% with per-allele OR of 1.30. For rarer variants of higher penetrance, the discovery stage has 80% power of detecting loci at P <1 × 10 −4 at MAF as low as 2% if the per-allele OR is at least 1.70. The entire sample (6,345 AMD cases and 15,980 controls) has 80% power to detect loci at P <5.0 × 10 −8 at MAF as low as 2% if the per-allele OR is at least 1.55 or at MAF as low as 9% with per-allele OR of 1.25, in line with the effect sizes being reported in this study. Supplementary Table 15A shows the power calculations to detect SNPs at the threshold of P <1 × 10 −4 in the discovery stage for bringing forward to the replication stage. Supplementary Table 15B shows the formal power calculations in the context of the combined discovery and replication stages. How to cite this article: Cheng, C.-Y. et al . New loci and coding variants confer risk for age-related macular degeneration in East Asians. Nat. Commun. 6:6063 doi: 10.1038/ncomms7063 (2015).